Stochastic signalling rewires the interaction map of a multiple feedback network during yeast evolution During evolution, genetic networks are rewired through strengthening or weakening their interactions to develop new regulatory schemes. In the galactose network, the GAL1 / GAL3 paralogues and the GAL2 gene enhance their own expression mediated by the Gal4p transcriptional activator. The wiring strength in these feedback loops is set by the number of Gal4p binding sites. Here we show using synthetic circuits that multiplying the binding sites increases the expression of a gene under the direct control of an activator, but this enhancement is not fed back in the circuit. The feedback loops are rather activated by genes that have frequent stochastic bursts and fast RNA decay rates. In this way, rapid adaptation to galactose can be triggered even by weakly expressed genes. Our results indicate that nonlinear stochastic transcriptional responses enable feedback loops to function autonomously, or contrary to what is dictated by the strength of interactions enclosing the circuit. The evolution of gene regulatory networks often relies on gene duplication and rewiring of regulatory links within a network [1] , [2] . The strength of gene regulatory interactions can be adjusted by the number and affinity of transcription factor binding sites in the gene regulatory regions [3] . When the interaction with a gene regulatory region is strengthened, the transcription factor is expected to have a stronger effect on its target gene. Accordingly, the strength of an interaction has been often equated with its functional importance. However, many regulatory motives, such as feedback loops, display nonlinear behaviour that is strongly affected by signalling patterns and stochasticity in gene expression [4] , [5] , [6] , [7] , [8] , [9] , [10] , [11] , which can modify the relevance of an interaction for a biological function. Little is known about how genetic regulatory elements and network interactions evolve to optimize the functioning of feedback loops [12] , [13] , [14] . The classical galactose regulatory network in Sacchromyces cerevisiae contains multiple feedback loops, which underlie the switch-like induction by galactose, control cellular memory, compensate gene dosage and reduce noise in gene expression [15] , [16] , [17] , [18] , [19] , [20] . Galactose is transported into the cells by Gal2p (ref. 21 ). In the earlier stages of evolution, a single bifunctional protein Gal1/3p catalysed the conversion of galactose and also transduced the information on the intracellular galactose concentration to the transcriptional circuitry, leading to the activation of the Gal4p transcriptional activator [22] , [23] , [24] . After gene duplication, paralogues typically undergo an asymmetric evolution, with one of them diverging slightly and the other considerably [25] . The more diverged Gal3p lost its enzymatic activity. Gal1p, on the other hand, is enzymatically active and retained a weak affinity to the signal transmission circuitry after the gene duplication event [22] , [26] . In this way, the GAL1 and GAL3 paralogues enclose parallel feedback circuitries and constitute the entry points to the catabolic and signalling cascades in the GAL regulon ( Fig. 1a ). The enzymatic branch encompassing Gal1p, Gal7p and Gal10p catabolizes galactose. The signalling pathway is composed of two consecutive inhibitory steps. Gal80p inhibits Gal4p; this inhibition is relieved when Gal80p itself becomes inhibited by Gal3p or Gal1p (ref. 21 ). 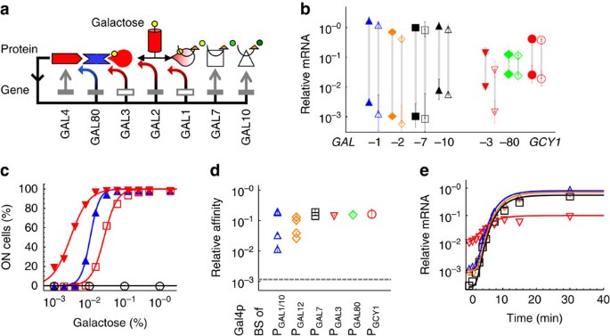Figure 1: Functional genomic comparison of the GAL regulatory regions. (a) Positive and negative feedback loops mediated by Gal4p are denoted by red and blue arrows. TheGAL1andGAL3paralogues are denoted by empty rectangles. (b) The minimal and maximal expression levels ofGALgenes were measured in wild-type (WT) cells grown for 5 h in raffinose medium with or without 0.5% galactose (filled symbols). To assess the dynamic range of gene expression in the presence of glucose (empty symbols), the minimal expression was measured in WT cells in 2% glucose; the maximal expression was measured in Δgal80, PGAL4-with-MutatedMig1pBS–GAL4cells. In these cells, the Gal4p maximally activates its target promoters, but glucose can directly reduce the expression of theGALgenes. Error bars indicate standard deviation,n=3. (c) Expression was induced for 5 h at the respective galactose concentrations in WT (blue triangles), Δgal1 (red squares), Δgal3 cells (black circles) and in cells in which highGAL1expression was driven constitutively by rtTA (red triangles). (d) The relative affinity corresponds to the ratio of maximally induced GFP expression driven by P[Gal4pBS]1-in-GAL1to that by PGAL1. A single Gal4p binding site (BS) from each of the indicated promoters was inserted into PGAL1-MMMMresulting in P[Gal4pBS]1-in-GAL1. PGAL1-MMMMis aGAL1promoter in which all four endogenous Gal4p binding sites are mutated. Error bars indicate standard deviation,n=3. The cellular background fluorescence is comparable to the fluorescence due to the PGAL1-MMMM–GFP construct (dashed line). (e) Induction kinetics of theGAL1(blue triangles),GAL2(orange diamonds),GAL3(red triangles) andGAL7(black squares) genes. The expression was induced by 0.5% galactose att=0 min. Figure 1: Functional genomic comparison of the GAL regulatory regions. ( a ) Positive and negative feedback loops mediated by Gal4p are denoted by red and blue arrows. The GAL1 and GAL3 paralogues are denoted by empty rectangles. ( b ) The minimal and maximal expression levels of GAL genes were measured in wild-type (WT) cells grown for 5 h in raffinose medium with or without 0.5% galactose (filled symbols). To assess the dynamic range of gene expression in the presence of glucose (empty symbols), the minimal expression was measured in WT cells in 2% glucose; the maximal expression was measured in Δgal80, P GAL4-with-MutatedMig1pBS – GAL4 cells. In these cells, the Gal4p maximally activates its target promoters, but glucose can directly reduce the expression of the GAL genes. Error bars indicate standard deviation, n= 3. ( c ) Expression was induced for 5 h at the respective galactose concentrations in WT (blue triangles), Δgal1 (red squares), Δgal3 cells (black circles) and in cells in which high GAL1 expression was driven constitutively by rtTA (red triangles). ( d ) The relative affinity corresponds to the ratio of maximally induced GFP expression driven by P [Gal4pBS]1-in-GAL1 to that by P GAL1 . A single Gal4p binding site (BS) from each of the indicated promoters was inserted into P GAL1-MMMM resulting in P [Gal4pBS]1-in-GAL1 . P GAL1-MMMM is a GAL1 promoter in which all four endogenous Gal4p binding sites are mutated. Error bars indicate standard deviation, n= 3. The cellular background fluorescence is comparable to the fluorescence due to the P GAL1-MMMM –GFP construct (dashed line). ( e ) Induction kinetics of the GAL1 (blue triangles), GAL2 (orange diamonds), GAL3 (red triangles) and GAL7 (black squares) genes. The expression was induced by 0.5% galactose at t =0 min. Full size image Similar to the evolution of the Gal1p and Gal3p proteins, their regulatory regions also evolved asymmetrically. GAL1 retained all four Gal4p binding sites, while GAL3 only one [22] . Here we studied how the divergence in gene regulatory regions affects the switching rate of positive feedback loops to the activated state. We found that strengthening the wiring of the circuit by increasing the number of activator binding sites in the autoregulatory promoter did not enhance the switching rate. This rate is rather determined by distribution of stochastic bursts, which is characteristic of each core promoter. This suggests that dynamical wiring—the network interactions to which the fluctuations in the network components direct the flow of signals—can override the affinity-based wiring maps. Strong dynamical wiring even enables weakly expressed genes, such as GAL3 when repressed by glucose, to activate the feedback loops efficiently. In comparison, its paralogue, GAL1 , has a weak dynamical wiring despite the strong interactions in the circuit. The GAL2 gene has both strong interactions and dynamical wiring. Feedback loops with strong dynamical wiring are targeted by the inhibitory signal elicited by glucose. High-affinity Gal4p binding sites in the GAL promoters Proteins that increase the intracellular concentration of galactose or enhance the activity of Gal4p enclose positive feedback loops, as exemplified by Gal2p and Gal3p (refs 16 and 18 ). Gal1p can, in principle, have two opposite effects. In the presence of galactose, Gal1p sequesters Gal80p, which leads to transcriptional activation by Gal4p ( Fig. 1a ). On the other hand, Gal1p catabolizes galactose, reducing its intracellular concentration, which affects Gal4p negatively. When GAL1 was constitutively overexpressed at a level comparable to the maximal galactose–induced expression level of the endogenous GAL1 ( Fig. 1b ), the activation of the network was enhanced ( Fig. 1c ). The deletion of GAL1 had the opposite effect ( Fig. 1c ), which indicates that the positive effect of GAL1 predominates. To see if promoters enclosing positive feedback loops ( GAL1 , -2 , -3 ) bear distinctive signatures, we measured the distribution of the affinities of Gal4p binding sites, the dynamic range and the kinetics of expression of the GAL promoters ( Fig. 1b,d,e ; Supplementary Fig. S1 ). Each promoter contains at least one high-affinity Gal4p binding site. Furthermore, there are at least two strong sites in promoters with multiple binding sites, which drive higher expression levels in galactose than those with a single site ( Fig. 1b,d ). The presence of two strong sites (for example, as in GAL7 ) is sufficient to drive maximally induced expression levels comparable to promoters with more than two sites, suggesting that the presence of additional weak sites adds only little further increments. These results indicate that it is the number rather than the affinity of the binding sites that is adjusted to set the maximal expression levels induced by galactose. Interestingly, promoters with single binding sites have higher basal expression than those with multiple binding sites ( Fig. 1b ). This elevated basal expression is not dependent on Gal4p ( Table 1 ), suggesting that the regulatory schemes that adjust the basal and maximal expression levels are distinct. Table 1 Ratios of the basal expression in wild-type (WT)/Δgal4 strains. Full size table In general, no common signature can be discerned for the promoters enclosing feedback loops. The GAL1 and GAL2 genes are functional homologues: they have multiple binding sites and a broad dynamical range. In contrast, the paralogue of GAL1 , GAL3 , has a single site and a narrow dynamic range ( Fig. 1b,d ). All of them follow rapid induction kinetics ( Fig. 1e ). Analysis of stochastic behaviour by synthetic circuits We performed stochastic simulations to assess how these two major determinants, the basal expression and the number of binding sites, affect the behaviour of a synthetic positive feedback loop ( Fig. 2 ). The resulting bimodal distribution of reporter gene expression displays a clear separation of ON and OFF peaks, that is, cell populations ( Fig. 2a,b ). As the GAL regulon is rapidly induced ( Fig. 1e ), we focused on short-term simulations and characterized the activation rate of the feedback loop by calculating the percentage of ON cells after 6 h (Methods). When the basal expression was raised from 0.003 to 0.03 mRNA copies per cell, the percentage of ON cells increased with linear proportionality ( Fig. 2c ). Similarly, increasing the number of the binding sites or the affinity of the activator enhanced the feedback activation ( Fig. 2a,b ). 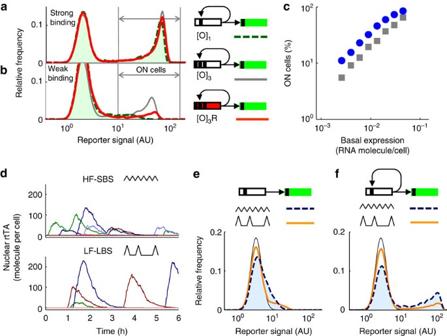Figure 2: Stochastic modelling of the feedback circuits. (a,b) Effect of the number of binding sites (black rectangles) and the refractory state (red box) in the feedback circuits. The green box denotes the reporter gene. The fluorescence distributions are shown for strong,KD=300 (a), and weak binding of the activator,KD=2,500 (b).KDis the dissociation constant. (c) The rate of basal transcription was varied betweenɛ=0.00026 and 0.0045 min−1, and the proportion of ON cells were calculated 6 h after induction atKD=200. The activator induced its own expression at a promoter withλ=3,γ=30 andμ=5 min−1; the mRNA decay rate of the activator, ΔRNA, was fixed at 0.2 min−1(grey squares). When ΔRNAwas doubled to 0.4 min−1(blue circles),μand the range ofɛwere also doubled to maintain the same mean expression levels. (d) Nuclear rtTA concentration trajectories are shown for ten runs of simulation (cells) in different colours. rtTA expression is driven promoters with low-frequency large burst-size (LF-LBS) and high-frequency small burst-size (HF-SBS) characteristics. (e,f) rtTA under the control of promoters with LF-LBS and HF-SBS characteristics (as labelled ind);KD=800. The green box denotes the reporter gene. The autoactivating promoter was characterized by the following parameters:λ=9,γ=30 andμ=5. While the mean value for the basal rtTA RNA levels was 0.02 molecules per cell for both direct control circuits, the ON percentages for the feedback circuits were 14% (LF-LBS) and 34% (HF-SBS). Figure 2: Stochastic modelling of the feedback circuits. ( a , b ) Effect of the number of binding sites (black rectangles) and the refractory state (red box) in the feedback circuits. The green box denotes the reporter gene. The fluorescence distributions are shown for strong, K D =300 ( a ), and weak binding of the activator, K D =2,500 ( b ). K D is the dissociation constant. ( c ) The rate of basal transcription was varied between ɛ =0.00026 and 0.0045 min −1 , and the proportion of ON cells were calculated 6 h after induction at K D =200. The activator induced its own expression at a promoter with λ =3, γ =30 and μ =5 min −1 ; the mRNA decay rate of the activator, Δ RNA , was fixed at 0.2 min −1 (grey squares). When Δ RNA was doubled to 0.4 min −1 (blue circles), μ and the range of ɛ were also doubled to maintain the same mean expression levels. ( d ) Nuclear rtTA concentration trajectories are shown for ten runs of simulation (cells) in different colours. rtTA expression is driven promoters with low-frequency large burst-size (LF-LBS) and high-frequency small burst-size (HF-SBS) characteristics. ( e , f ) rtTA under the control of promoters with LF-LBS and HF-SBS characteristics (as labelled in d ); K D =800. The green box denotes the reporter gene. The autoactivating promoter was characterized by the following parameters: λ =9, γ =30 and μ =5. While the mean value for the basal rtTA RNA levels was 0.02 molecules per cell for both direct control circuits, the ON percentages for the feedback circuits were 14% (LF-LBS) and 34% (HF-SBS). Full size image We tested the above predictions using gene circuits incorporating the synthetic activator, rtTA ( Fig. 3a ), which is a fusion protein of the bacterial DNA binding domain (DBD) TetR and the viral transcriptional activation domain VP16. With the help of this activator, the role of gene regulatory sequences in feedback loops can be assessed independently, without the interference from the GAL network. In the feedback constructs, tet operators were inserted into the GAL promoters to drive rtTA expression retroactively (P [tetO]-in-GAL –rtTA, Supplementary Fig. S1 ). 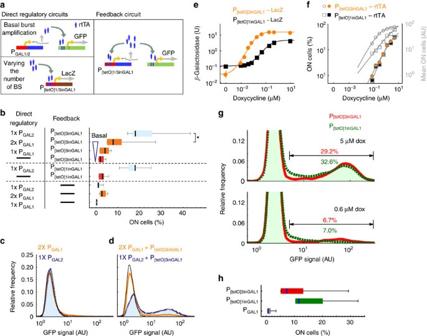Figure 3: Direct and retroactive effects in synthetic gene circuits. (a) Schemes of the synthetic gene circuits. BS stands for binding sites. (b) The role of basal expression in the direct and feedback circuits. Cells containing different combinations of these rtTA circuits were induced with 5 μM doxycycline (dox) for 6 h, in glycerol medium. The black bar in a box indicates the median of the ON cell percentage; the margins of a box indicate the first and third quartiles; whiskers indicate the data range. *P=0.015 for Mann–Whitney test for the median,n=7. (c,d) The distribution of GFP fluorescence signal when rtTA was driven by the basal expression of PGAL1(orange lines, kurtosis=7.04) or PGAL2(blue dashed lines, kurtosis=2.84). One representative experiment frombis shown. The black lines denote the cellular autofluorescence. (e) The direct effect of the number of activator binding sites. The reporter lacZ under P[tetO]1-in-GAL1or P[tetO]3-in-GAL1was activated by constitutively expressed rtTA. (f–h) The retroactive effect of the number of activator binding sites. P[tetO]1-in-GAL1and P[tetO]3-in-GAL1feedback circuits were activated with doxycycline in raffinose medium for 6 h. (f) The percentage and the mean fluorescence of the ON cells. (g) The GFP fluorescence distribution of the cells containing the P[tetO]1-in-GAL1–rtTA (green dashed lines) and P[tetO]3-in-GAL1–rtTA (red lines) constructs was measured at high and intermediate doxycycline concentrations. (h) The ON cell percentages measured at 5 μM doxycycline; displayed as inb,n=6. Figure 3: Direct and retroactive effects in synthetic gene circuits. ( a ) Schemes of the synthetic gene circuits. BS stands for binding sites. ( b ) The role of basal expression in the direct and feedback circuits. Cells containing different combinations of these rtTA circuits were induced with 5 μM doxycycline (dox) for 6 h, in glycerol medium. The black bar in a box indicates the median of the ON cell percentage; the margins of a box indicate the first and third quartiles; whiskers indicate the data range. * P= 0.015 for Mann–Whitney test for the median, n =7. ( c , d ) The distribution of GFP fluorescence signal when rtTA was driven by the basal expression of P GAL1 (orange lines, kurtosis=7.04) or P GAL2 (blue dashed lines, kurtosis=2.84). One representative experiment from b is shown. The black lines denote the cellular autofluorescence. ( e ) The direct effect of the number of activator binding sites. The reporter lacZ under P [tetO]1-in-GAL1 or P [tetO]3-in-GAL1 was activated by constitutively expressed rtTA. ( f – h ) The retroactive effect of the number of activator binding sites. P [tetO]1-in-GAL1 and P [tetO]3-in-GAL1 feedback circuits were activated with doxycycline in raffinose medium for 6 h. ( f ) The percentage and the mean fluorescence of the ON cells. ( g ) The GFP fluorescence distribution of the cells containing the P [tetO]1-in-GAL1 –rtTA (green dashed lines) and P [tetO]3-in-GAL1 –rtTA (red lines) constructs was measured at high and intermediate doxycycline concentrations. ( h ) The ON cell percentages measured at 5 μM doxycycline; displayed as in b , n =6. Full size image Two types of control circuits were designed to assess the role of basal expression and the number of binding sites in the context of direct regulation ( Fig. 3a ). When a GAL promoter drives the expression of rtTA (P GAL –rtTA) in Δgal4 strains, the basal expression of the GAL promoter is amplified and read out by a P tet –GFP (green fluorescent protein) reporter construct at the single cell level. When P [tetO]-in-GAL drives the expression of a reporter gene directly, the effect of varying the number of activator binding sites ( tet operators) can be studied. In this case, gene expression is not amplified; therefore, the more sensitive lacZ reporter was used to reliably assess low expression levels. In all constructs, the affinity of rtTA to the tet operators was adjusted by doxycycline [27] . Dynamical wiring of circuits by stochastic bursting The contribution of the basal expression to the activation of the feedback loops was examined by adding P GAL1 –rtTA direct regulatory constructs to a single-copy P [tetO]3-in-GAL1 –rtTA feedback construct. As the copy number of genes providing basal expression was raised from one to three, the percentage of ON cells increased proportionally ( Fig. 3b ). As GAL1 and GAL2 have similar low basal expression levels ( Fig. 1c ), they are expected to trigger similar weak responses. Interestingly, the shape of the GFP distributions differed in the respective direct regulatory circuits. It was narrow and symmetric for P GAL2 –rtTA, while P GAL1 –rtTA drove high GFP expression levels in few cells, resulting in a distribution with a long right tail ( Fig. 3c ). The basal expression of these genes is low; at most one mRNA molecule is produced in 2 h, on average. This slow bursting can be faithfully amplified by the direct regulatory circuit given its components decay with a half-life of around 10 min (Methods). If a single mRNA is produced at each round of promoter activation, multiple small nuclear rtTA concentration bursts are predicted to arise in a cell population ( Fig. 2d ). The resulting distribution of the reporter gene is comparable to that of GAL2 ( Figs 2e and 3c ). If the frequency of promoter activation is lower, but gene expression is compensated by producing multiple RNA molecules at each round, the distribution is predicted to be more asymmetric, comparable to that seen for GAL1 ( Figs 2e and 3c ). When the respective bursting kinetics drove the positive feedback loops, a twofold reduction in the percentage of ON cells was predicted with respect to the frequent small bursting, even though the mean values of their basal expression were identical ( Fig. 2f ). To verify the above predictions, the P [tetO]3-in-GAL1 –rtTA feedback circuit was supplemented with a single-copy P GAL2 –rtTA. This led to a significantly stronger boost in generating ON cells than addition of even a two-copy P GAL1 –rtTA ( Fig. 3b,d ). This confirms that equal mean basal expression levels with different bursting kinetics result in considerable differences in the speed of feedback loop activation. Counteraction of multiple binding sites Next, we studied how the number of activator binding sites affects the feedback. As the number of high-affinity Gal4p binding sites is the major determinant of gene expression in the GAL regulon, we inserted single or multiple high-affinity tet operators into the GAL1 promoter. The response in the direct regulatory circuit was stronger for the promoter with three operators ( Fig. 3e ). However, no difference was observed in the percentage of ON cells generated by the P [tetO]1-in-GAL1 –rtTA and P [tetO]3-in-GAL1 –rtTA feedback constructs at the entire range of doxycycline concentration ( Fig. 3b,f–h ); only the mean expression level of the ON cells was higher for the construct with multiple operators at low doxycycline concentration ( Fig. 3f,g ). This stands in contrast to the simulations, which predict that at weak activator binding, the percentage of ON cells is higher for constructs with multiple operators ( Fig. 2b ). To explain this discrepancy, we have taken into account previous observations revealing that promoters with multiple operators have lower relative activation rates, possibly due to a refractory state between the transcriptional bursts [4] , [28] , [29] . The parameters of the refractory state were adjusted so that the simulations reproduce the mean features of the direct response of the P [tetO]3-in-GAL1 –reporter construct: the higher maximal expression and steeper convergence to zero at low induction in comparison to the P [tetO]1-in-GAL1 –reporter construct ( Fig. 3e ; Supplementary Fig. S2 ). Next, we simulated how this refractory state affected the activation of the feedback circuit. When the binding of the activator to promoter was weak, the refractory state reduced the ON peak without affecting its mean value, similar to the experimental observations ( Figs 2b and 3g ). At strong binding, the distribution was not affected by the refractory state ( Fig. 2a ). The experiments also revealed that the basal expression of P [tetO]3-in-GAL1 –reporter is, counterintuitively, lower than that of the P [tetO]1-in-GAL1 –reporter, which may also reflect another effect of the refractory state ( Fig. 3e ) [27] . This reduced basal expression is expected to contribute to the weakening of the activation of the feedback loop driven by multiple binding sites ( Fig. 2c ). The above findings using synthetic circuits reveal that the multiple binding sites do not compensate the low basal expression of GAL1 to activate the feedback loop. Rather, it is further debilitated by the low-frequency bursting kinetics ( Figs 2e and 3c,d ). Having few Gal4p binding sites accelerates adaptation We tested if the mechanisms that weaken the retroactive effect of GAL1 manifest themselves in the context of the endogenous GAL network, as well. When the GAL1 promoter drove the expression of the GAL3 gene, the activation of the network in response to galactose was very slow, confirming the above results with the synthetic circuits ( Fig. 4a ). Surprisingly, when only a single high-affinity Gal4p binding site was retained in the GAL1 promoter, P [Gal4pBS]1-in-GAL1 , the response showed an approximately threefold enhancement ( Fig. 4a ). The fact that the reduction of binding site number did not weaken the response is consistent with the results on the synthetic circuits. Moreover, the surprisingly strong enhancement points to additional mechanisms specific for Gal4p. Indeed, the basal expression increased nearly ten times when the number of binding sites was reduced to one ( Fig. 4b ). Having the other binding sites mutated did not increase basal expression on its own ( Fig. 1d ). It has been suggested that the Gal4p bound to multiple sites can be more efficiently inhibited by Gal80p, lowering the basal expression in comparison to promoters with a single site [30] . 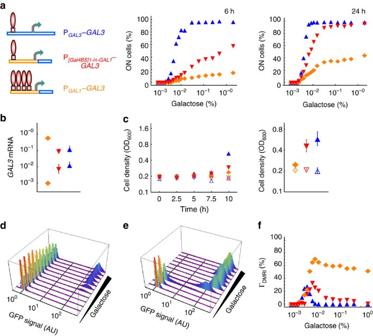Figure 4: Retroactive effects on the cellular memory. The activity of the GAL network was read out by a PGAL1–GFP reporter in strains where the PGAL1(orange diamonds), P[Gal4pBS]1-in-GAL1(red triangles) or the PGAL3(blue triangles) promoters drove theGAL3expression. (a) The percentage of ON cells was measured 6 and 24 h after the induction by the respective galactose concentrations. (b)GAL3mRNA levels driven by the indicated promoters. Minimal expression was measured in cells grown in raffinose medium (bottom symbol), while maximal expression was induced by 0.5% galactose in cells with galactose history (top symbols). (c) Cell density was measured after inoculating cells into the glycerol medium without galactose (empty symbols) or in the presence of 0.1% galactose (filled symbols). The right panel shows the mean±s.d. of the cell density measured after 10 h,n=3. (d,e) The GFP fluorescence distribution of PGAL1–GAL3cells is shown 24 h after inducing cells with raffinose (d) or galactose (e) histories at the respective galactose concentrations. (f) The 24-h memory indices are shown. Figure 4: Retroactive effects on the cellular memory. The activity of the GAL network was read out by a P GAL1 –GFP reporter in strains where the P GAL1 (orange diamonds), P [Gal4pBS]1-in-GAL1 (red triangles) or the P GAL3 (blue triangles) promoters drove the GAL3 expression. ( a ) The percentage of ON cells was measured 6 and 24 h after the induction by the respective galactose concentrations. ( b ) GAL3 mRNA levels driven by the indicated promoters. Minimal expression was measured in cells grown in raffinose medium (bottom symbol), while maximal expression was induced by 0.5% galactose in cells with galactose history (top symbols). ( c ) Cell density was measured after inoculating cells into the glycerol medium without galactose (empty symbols) or in the presence of 0.1% galactose (filled symbols). The right panel shows the mean±s.d. of the cell density measured after 10 h, n =3. ( d , e ) The GFP fluorescence distribution of P GAL1 – GAL3 cells is shown 24 h after inducing cells with raffinose ( d ) or galactose ( e ) histories at the respective galactose concentrations. ( f ) The 24-h memory indices are shown. Full size image The GAL1 promoter with a single Gal4p binding site has a dynamic range of expression comparable to that of GAL3 ( Fig. 4b ). However, its switching rate is still considerably slower than that of the wild-type GAL3 promoter ( Fig. 4a ), which is likely to reflect the slow bursting kinetics of the GAL1 core promoter evidenced in synthetic circuits. Thus, P [Gal4pBS]1-in-GAL1 , which can be considered as an evolutionary intermediate between P GAL1 and P GAL3 , recapitulates all the phenomena observed for the synthetic feedback circuits enclosed by the P [tetO]1-in-GAL1 promoter. We tested if the expression of these constructs impacts on cellular fitness. The growth rates on addition of galactose to the culture recapitulated the differences in the speed of network activation in the respective strains ( Fig. 4a ), that is, the following order was observed: P GAL3 >P [Gal4pBS]1-in-GAL1 >P GAL1 ( Fig. 4c ). When the entire cell population switched to the ON state, we reduced the galactose concentration to measure how quickly the system returns to the OFF state. This deactivation rate was rather uniform for all strains. This implies that cellular memory—defined as the difference between the ON cell percentages measured in cultures that were preincubated with or without 0.5% galactose ( Fig. 4d,e )—is largely determined by the switching rate to the ON state. Thus, the memory index decreases in the following order: P GAL1 >P [Gal4pBS]1-in-GAL1 >P GAL3 ( Fig. 4f ). This suggests that it is the adaptation speed and fitness rather than cellular memory that are optimized by the promoter of the GAL3 gene. Strongly retroactive genes produce short half-life mRNAs Gene expression, and hence the functioning of the feedback loop, is jointly determined by mRNA production and decay rates. If both these rates are doubled for an mRNA encoding an activator in a positive feedback loop, its mean expression level does not change; however, a stochastic simulation reveals that more ON cells are produced ( Fig. 2c ). Interestingly, the GAL1 mRNA decays slowly in comparison to the GAL2 mRNA on removal of galactose ( Fig. 5a ), suggesting that the retroactive effect of GAL1 is not weakened only by slow bursting but also by having slower mRNA production and decay rates than its functional genomic counterpart with equal dynamic range, GAL2 . The decay of GAL2 and GAL3 mRNA was faster than that of GAL1 , also in the presence of glucose ( Fig. 5b ). 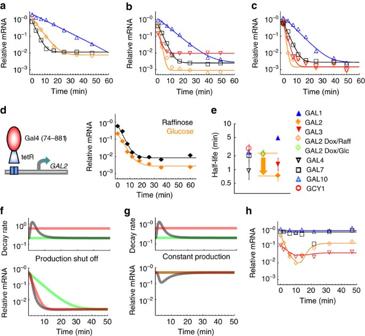Figure 5: RNA decay rates in the GAL regulon. (a) The following RNA half-lives were fit from the measurements after washing out galactose.GAL1=8.1 min (blue triangles),GAL2=3 min (orange diamonds) andGAL7=1.7 min (black squares). (b,c) RNA decay is measured after addition of 2% glucose to wild-type (b) and PGAL1–GAL3(c) cells that had been induced by 0.02% galactose in raffinose medium. For theGAL3mRNA (red triangles), the half-life was 1.3 min when driven by the wild-type promoter and 1.2 min when driven by PGAL1; forGAL1=4 min (blue triangles),GAL2=0.6 min (orange diamonds) andGAL7=1.77 min (black squares). (d) TheGAL2mRNA decay was measured after adding 2 μM doxycycline to dissociate the TetR–Gal4AD from thetetoperators inserted into theGAL2promoter. Half-lives of 2.33±0.39 and 2.23±0.31 min were fitted for cells cultured in raffinose (black) and glucose (orange) media, respectively. (e) Mean RNA half-lives were fitted from experiments shown inbandd. Error bars indicate standard deviation,n=3. The difference between the half-lives for theGAL2mRNA measured inbanddis denoted by a yellow arrow. (f,g) Top panels: the default value of RNA decay rate (green line) was increased transiently (grey line) or constantly (red line). Bottom panels: the corresponding RNA levels were calculated. For the red curves, higher production rates were used to compensate the faster decay. (f) The RNA production rate is reduced to a baseline level att=0 min. The resulting RNA decay curves with transiently and constantly elevated decay rates are very similar. (g) With constant production rates, the level of RNA with time varying decay rate (grey curve) is clearly distinguished from those with constant decay rates (overlapping red and green lines). (h) RNA levels measured after adding 2% glucose to Δgal80, PGAL4-with-MutatedMig1pBS–GAL4cells att=0 min. The cells were precultured in raffinose medium. Symbols of the genes are indicated as inb. Figure 5: RNA decay rates in the GAL regulon. ( a ) The following RNA half-lives were fit from the measurements after washing out galactose. GAL1 =8.1 min (blue triangles), GAL2 =3 min (orange diamonds) and GAL7 =1.7 min (black squares). ( b , c ) RNA decay is measured after addition of 2% glucose to wild-type ( b ) and P GAL1 – GAL3 ( c ) cells that had been induced by 0.02% galactose in raffinose medium. For the GAL3 mRNA (red triangles), the half-life was 1.3 min when driven by the wild-type promoter and 1.2 min when driven by P GAL1 ; for GAL1 =4 min (blue triangles), GAL2 =0.6 min (orange diamonds) and GAL7 =1.77 min (black squares). ( d ) The GAL2 mRNA decay was measured after adding 2 μM doxycycline to dissociate the TetR–Gal4AD from the tet operators inserted into the GAL2 promoter. Half-lives of 2.33±0.39 and 2.23±0.31 min were fitted for cells cultured in raffinose (black) and glucose (orange) media, respectively. ( e ) Mean RNA half-lives were fitted from experiments shown in b and d . Error bars indicate standard deviation, n= 3. The difference between the half-lives for the GAL2 mRNA measured in b and d is denoted by a yellow arrow. ( f , g ) Top panels: the default value of RNA decay rate (green line) was increased transiently (grey line) or constantly (red line). Bottom panels: the corresponding RNA levels were calculated. For the red curves, higher production rates were used to compensate the faster decay. ( f ) The RNA production rate is reduced to a baseline level at t =0 min. The resulting RNA decay curves with transiently and constantly elevated decay rates are very similar. ( g ) With constant production rates, the level of RNA with time varying decay rate (grey curve) is clearly distinguished from those with constant decay rates (overlapping red and green lines). ( h ) RNA levels measured after adding 2% glucose to Δgal80, P GAL4-with-MutatedMig1pBS – GAL4 cells at t =0 min. The cells were precultured in raffinose medium. Symbols of the genes are indicated as in b . Full size image Strongly retroactive genes are inhibited by glucose Next, we studied the deactivation of the GAL network by glucose ( Fig. 5b–h ) [31] . The transcriptional inhibition of the GAL regulon by glucose is mediated by two proteins: Gal80p and the Mig1p repressor. As Mig1p represses GAL4 , both these pathways converge on Gal4p (refs 32 and 33 ). Thus, the Gal4p-independent effects of glucose on GAL genes can be discerned by measuring their expression in Δgal80 cells, in which the Mig1p sites in P GAL4 are also mutated (P GAL4-with-MutatedMig1pBS – GAL4 ). Among the GAL genes, it was only GAL3 whose expression was significantly repressed by glucose in these cells ( Fig. 1b ). This suggests that repression of GAL3 by glucose is used to adjust the activity of the GAL signalling pathway. Interestingly, the percentage of ON cells in glucose containing media was higher for wild-type cells than for P GAL1 – GAL3 cells, even though both of them drove similar GAL3 expression levels ( Supplementary Fig. S3 ). The differential activation of the GAL3 loop in these cells may be due to the different bursting kinetics of the GAL1 and GAL3 promoters. Indeed, the amplification of GAL3 basal bursts in the direct regulatory circuit results in a distribution similar to that of GAL2 ( Fig. 6 ). Thus, this bursting is likely to enable the GAL3 promoter to generate ON cells even when repressed by intermediate glucose concentrations. 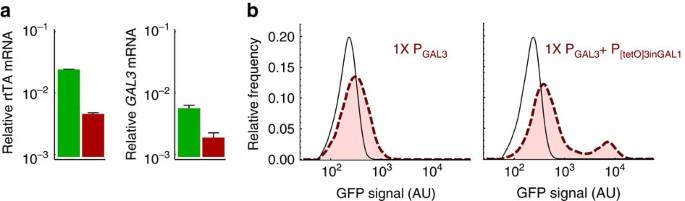Figure 6: Retroactive effect of theGAL3promoter in the presence of glucose. (a) The cells containing a one-copy PGAL3–rtTA direct regulatory circuit were grown in raffinose medium (green) or in raffinose medium with 0.32% glucose (red) for both the overnight preculturing and the subsequent 6-h growth period, following which RNA was isolated. Error bars indicate standard deviation,n=3. (b) Cells containing either the direct regulatory circuit PGAL3–rtTA (left panel) or the feedback circuit with P[tetO]3-in-GAL1–rtTA activated by PGAL3–rtTA (right panel) were grown overnight in raffinose medium with 0.32% glucose. Subsequently, the cells were induced by 5 μM doxycycline for 6 h in the same medium (dark red dashed lines) and GFP fluorescence was measured. The black lines denote the cellular autofluorescence. The kurtosis for the background distribution is 0.56 and for the direct regulatory circuit is −0.07. Figure 6: Retroactive effect of the GAL3 promoter in the presence of glucose. ( a ) The cells containing a one-copy P GAL3 –rtTA direct regulatory circuit were grown in raffinose medium (green) or in raffinose medium with 0.32% glucose (red) for both the overnight preculturing and the subsequent 6-h growth period, following which RNA was isolated. Error bars indicate standard deviation, n= 3. ( b ) Cells containing either the direct regulatory circuit P GAL3 –rtTA (left panel) or the feedback circuit with P [tetO]3-in-GAL1 –rtTA activated by P GAL3 –rtTA (right panel) were grown overnight in raffinose medium with 0.32% glucose. Subsequently, the cells were induced by 5 μM doxycycline for 6 h in the same medium (dark red dashed lines) and GFP fluorescence was measured. The black lines denote the cellular autofluorescence. The kurtosis for the background distribution is 0.56 and for the direct regulatory circuit is −0.07. Full size image The decay of the GAL3 mRNA is fast ( Fig. 5b ). The fast decay is preserved even when its promoter is replaced by P GAL1 ( Fig. 5c ). This suggests that the fast decay is not due to the 5′UTR region of GAL3 , and that the evolution of gene regulatory regions after the gene duplication event has not been restricted to the promoter alone. Unlike GAL3 , GAL2 is not sensitive to glucose when the signal transmission through Gal4p is interrupted ( Fig. 1b ). Yet the decay of GAL2 mRNA accelerated around four times on exposure of cells to glucose, with respect to the decay rate measured on removal of galactose ( Fig. 5a,b ). Such an acceleration of the decay was not observed when transcription was shut off by dissociating a chimerical TetR–Gal4AD activator from the GAL2 promoter on addition of doxycycline ( Fig. 5d,e ). In this experiment, glucose has been present continuously. Thus, the above contradictory observations may be reconciled with the hypothesis that glucose destabilizes the GAL2 mRNAs only transiently, increasing the RNA decay rates for a short time immediately after the cells had been exposed to glucose. The simulations reveal that when the same signal is responsible for both shutting off transcription and accelerating the decay it is difficult to discern whether the elevation of the decay rate is constant or transient ( Fig. 5f ). A distinction of the two mechanisms can be attained with the help of mutants where the signal only influences the decay but does not shut off transcription ( Fig. 5g ). Indeed, in the genetic background where glucose cannot shut off transcription through Gal4p (ref. 33 ), the GAL2 mRNA level was selectively reduced for a short period of time and rebounded afterward ( Fig. 5h ). This reduction in mRNA level may synergize with the glucose-induced degradation of the Gal2p protein [34] . Positive feedback has been thought to follow the dictates of direct promoter responses. We have identified, however, determinants in the GAL regulon that enable the same gene regulatory region to respond differently to a signal depending on whether it propagates directly or retroactively ( Fig. 7 ). With the help of synthetic circuits we showed that stochastic signalling mechanisms can tune the activation of feedback loops without the need to change the mean level of the basal expression. While GAL1 has a weak retroactive effect, its functional genomic homolog GAL2 and its paralogue GAL3 have strong retroactive effect due their high-frequency small-sized stochastic bursts in basal expression. On the other hand, having only a single activator binding site in GAL3 does not prevent its efficient retroactive activation even in glucose, as the reduction of binding sites is compensated by the alleviation of a stochastic refractory state. 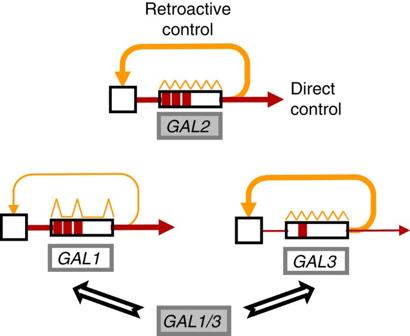Figure 7: Genetic determinants of direct and retroactive effects. The direct effect is proportional to the number of Gal4 binding sites.GAL2andGAL3modulate gene expression by high-frequency low-size bursting, which boosts the retroactive effect. Furthermore, the reduction of Gal4p binding sites inGAL3enhances the retroactive effect due to a weakened refractory state and the concomitant increase in basal expression. Figure 7: Genetic determinants of direct and retroactive effects. The direct effect is proportional to the number of Gal4 binding sites. GAL2 and GAL3 modulate gene expression by high-frequency low-size bursting, which boosts the retroactive effect. Furthermore, the reduction of Gal4p binding sites in GAL3 enhances the retroactive effect due to a weakened refractory state and the concomitant increase in basal expression. Full size image The specific ability of Gal4p to increase basal expression due to the reduction of binding sites [30] ( Fig. 4b ) is overshadowed in the GAL3 promoter by the elevated Gal4-independent basal expression ( Fig. 1b , Table 1 ). Therefore, this ability of Gal4p is not used to boost the GAL3 feedback activation in the current yeast genome, but it may have had a role in the early stages of evolution after the GAL1/3 gene duplication. Interestingly, genes that have strong retroactive response to galactose are targeted by the inhibitory effect of glucose. The transient acceleration of GAL2 mRNA decay may serve to rapidly deactivate the GAL2 feedback on exposure of cells to glucose. On the other hand, the constant inhibition of GAL3 expression may serve to adjust the steady-state activation of the GAL3 , according to the ratio of galactose to glucose concentration. It is unclear whether protein networks are also capable of directing information flow by differential enhancement of the direct or the retroactive effects. Nonlinear stochastic phenomena—on which the separation of these effects relies—arise prominently at the level of gene regulation rather than at the level of protein interactions [28] , [29] , [35] . This may render gene expression superior in its ability of control signalling by dynamical wiring ( Fig. 7 ). It has been reported that it is difficult to predict gene expression based on evolutionary changes in the DNA sequence [36] . Our results indicate that even knowing expression levels is not sufficient to predict the retroactive effects. Synthetic circuits offer a convenient means to assess the relative strengths of direct and retroactive effects of a gene regulatory element. Mapping the strength of such functional interactions is of paramount importance, as this dynamical wiring may not follow or may even contradict the logic of network topology relying on interaction strengths between network components. Yeast strains and genetic constructs The yeast strains are described in Supplementary Tables S1–S3 . All genetic constructs were integrated into the chromosome. For the synthetic feedback constructs, minimal possible pleiotropic effects were desired; therefore, we used the fully synthetic rtTA (rTetR–VP16) activator [27] . Conversely, it was important for the RNA decay measurements that the GAL2 mRNA is induced by the endogenous transcriptional mechanisms. Therefore, we used the TetR–Gal4AD transcriptional activator, which was obtained by fusing tetR through a linker VAAG peptide to a Gal4p fragment comprising the C-terminal amino acids 74–881 (Gal4AD). TetR serves as the DBD, while Gal4p(74–881) lacks the Gal4 DBD and serves as an activation domain. Growth conditions Cells were aerobically cultured at 30 °C in minimal drop out medium (typically URA, because our reporter gene is with pRS306) supplemented with carbon sources as indicated. Galactose activates while glucose represses the GAL regulon. For control experiments, raffinose or glycerol was used as supplement. The raffinose medium refers to a minimal medium with 2% filter-sterilized raffinose supplemented with 0.005% glucose. For growth in glycerol medium, the cells were cultured overnight in a raffinose medium, washed and diluted to a density of OD 600 =0.2 in glycerol medium, which refers to a minimal medium with 3% glycerol as the mere carbon source. This medium supported only a very slow cellular growth. To induce the synthetic circuits in the glycerol medium, doxycycline was added at the indicated concentrations after overnight preincubation in raffinose medium, and cells were incubated for further 6 h in glycerol medium before cytometry. To measure fitness in glycerol, cells with the different GAL3 expression constructs were grown for 10 h in glycerol medium with or without 0.1% galactose. OD 600 was then recorded. β-Galactosidase assay The expression of the lacZ gene was measured using chlorophenol red- β -galactopyranoside as a substrate for the β -galactosidase. Briefly, the cells were induced by doxycycline for 6 h in raffinose medium. Cells were then pelleted, washed and resuspended with 100 μl buffer 1 (100 mM HEPES; 154 mM NaCl; 4.5 mM L -aspartate hemi Mg; 1% bovine serum albumin; 0.05% (v/v) Tween 20; pH=7.30). The cells were disrupted by two freeze/thaw cycles using liquid nitrogen, following which 700 μl ice-cold buffer 1 containing 2.23 mM chlorophenol red- β -galactopyranoside was added. The colour development was started on incubation at 37 °C. The reaction was stopped by adding 300 μl of 3 mM ZnCl 2 . After removal of cell debris, the OD 578 of the supernatant was recorded. The β-galactosidase unit is defined as 1,000×OD 578 /[development time (min)×cell density (OD 600 )]. RNA measurements Samples (1.5 ml) of the culture with a cell density of OD 600 =0.7–1.5 were taken at different time points and snap-frozen with liquid nitrogen. The RNA was isolated with the RiboPure Kit (Ambion) and the complementary DNA was synthesized with a mixture of random and oligo-dT primers (QuantiTect Reverse Transcription Kit). The real-time quantitative PCR was performed with KAPA SYBR FAST qPCR Kit (Kapa Biosystems) using an ABI 7900HT detection system (Applied Biosystems). The primers used for the amplification are listed in the Supplementary Table S4 . All RNA values are normalized by ACT1 RNA. RNA decay measurements The decay rate was fit assuming an exponential decay with a residual expression. To measure the mRNA degradation after galactose removal, the cells were cultured overnight in a medium supplied with 0.5% galactose. Afterwards, the cells were transferred to a fresh medium containing 0.1% galactose and incubated for further 4 h. At t =0, the medium was replaced by raffinose medium. Memory experiments The cells were inoculated at a cell density of OD 600 =10 −8 and grown up to OD 600 =1 in raffinose medium without or with 0.5% galactose to obtain cells with raffinose and galactose histories, respectively. Cells were then washed and inoculated into a medium at OD 600 =0.1, containing an appropriate concentration of galactose (0.001–2%) and grown for 6–24 h. For the flow cytometry measurements, the cell density was between OD 600 =0.2–0.8. The memory index, Γ MRI was defined as the difference of probability distributions arising from the no-induction and high-induction histories [37] . A discretized version of this definition relies on the peaks, so that Γ DMRI equals the difference of the percentage of ON cells found in the populations with induction and no-induction histories. Flow cytometry and analysis of cell fluorescence distributions GFP fluorescence (FL) was measured by Beckman Coulter FC500 cytometer using the 488 nm laser and the 520 nm band-pass emission filter, coupled to a 550 nm long-pass dichroic mirror. Gating based on the forward- and side-scatter signal was performed to omit the cell debris and clusters. At least 10,000 cell events were recorded for a single measurement [38] . To measure the ON cell percentage, a threshold was set each time to optimize the separation of the two populations in the GFP bimodal distribution; subsequently, the proportion of cells above this threshold was calculated. To characterize the tails of the distribution of cellular GFP FL, the kurtosis was calculated based on the fourth moment of single-cell florescence values x i =Log 10 FL i where [xmacr] is the corresponding mean value for a population consisting of n cells: A normally distributed x i results in a kurtosis value of 0 and distributions with long tales have large positive values. Stochastic simulation of the reactions The stochastic simulations of the reactions occurring in the synthetic circuits were performed in MATLAB using the Gillespie algorithm [39] . The posttranscriptional processes were described by reaction rates with linear dependence on reactant concentrations, whereas the occupancy ( Occ ) of the promoter by rtTA was described by a rapid equilibrium process: The transition rate of the promoter from an inactive state I to an active state, A , is calculated by multiplying Occ and the promoter activation rate constant, λ . Accordingly, this transition has a hyperbolic dependence on rtTA concentration. The reverse transition occurs at a rate of γA . RNA is produced from the active promoter with a rate of μA . The basal mRNA transcription was described by simple birth process with a rate constant ɛ . Thus, the mean values for the rtTA induced and basal RNA expression level are given by and The parameter values of the reactions ( Supplementary Table S5 ) are based on previous measurements [4] , [40] , [41] . Calculation of cellular GFP FL Cellular FL is composed of background and GFP FL. Therefore, values representing the concentration of background chemical entities were sampled from a log-normal distribution with a mean μ LN and standard deviation σ LN , and were added to the calculated GFP molecule numbers. The resulting sum was divided by 500 to convert molecule number into FL intensity (AU). μ LN =7 and σ LN =0.25; and μ LN =7.4 and σ LN =0.35 were taken for simulations to imitate cellular background FL in raffinose and glycerol, respectively. ON cells were defined as runs with a reporter signal higher than 10 AU. Stochastic bursting in the basal transcription The high-frequency small burst-size promoter produces a single RNA molecule at a frequency of ɛ =0.002 min −1 . In contrast, the low-frequency large burst-size promoter fires at a frequency of ɛ =0.0005 min −1 and produces variable numbers of RNA that follows a Poissonian distribution with a mean of ν =4. In this way, both promoters produce the same amount of mRNA molecules on average. The production of mRNA by low-frequency large burst-size promoter corresponds to a mechanism when a rarely bursting promoter enters an open configuration for a short period of time and the occurrence of mRNA transcription is a random process [42] . Stochastic modelling of the refractory state of promoters The positive feedback circuit with one and three tet operators was examined in raffinose medium. To simulate the tripling of the association rate due to tripling of the binding sites, λ =3 for [O] 1 was increased to λ =9 for [O] 3 ; and γ =10, μ =5 and ɛ =0.002 min −1 were kept constant. To simulate the refractory state in promoters with multiple binding sites, we assumed that this state persists when the promoter is inactive and peters out after the first transcriptional burst is induced by rtTA. Thus, the refractory state wields its influence during the early stages of the simulated transcriptional induction. After induction, the first round of rtTA-induced mRNA transcription is accompanied by the production of transcriptional inhibitory molecules ( N inh =10). The inhibitory molecules decay at a rate of deact =0.02 min −1 . The inhibitor decreases the frequency of promoter activation by regulating the permissive state. The refractory state vanishes at a speed proportional to the bound activator, while the inhibitor enhances the formation of the refractory state [38] . Thus, the rate of activation of a refractory promoter is given by: with α= 0.001 and β =0.2. We studied the behaviour of a refractory promoter with three operators [O] 3R by comparing it to promoters with one [O] 1 and three [O] 3 operators. To assess the behaviour of a [O] 3R –reporter construct in a direct control circuit driven by rtTA, the concentration of rtTA was adjusted to reflect the parameters of the P CLN3 –rtTA construct: the mean concentration of the rtTA mRNA and the nuclear rtTA protein was 0.4 and 104 copy per cell, respectively. How to cite this article: Hsu, C. et al . Stochastic signalling rewires the interaction map of a multiple feedback network during yeast evolution. Nat. Commun. 3:682 doi: 10.1038/ncomms1687 (2012).